Implementation of a quantum metamaterial using superconducting qubits The key issue for the implementation of a metamaterial is to demonstrate the existence of collective modes corresponding to coherent oscillations of the meta-atoms. Atoms of natural materials interact with electromagnetic fields as quantum two-level systems. Artificial quantum two-level systems can be made, for example, using superconducting nonlinear resonators cooled down to their ground state. Here we perform an experiment in which 20 of these quantum meta-atoms, so-called flux qubits, are embedded into a microwave resonator. We observe the dispersive shift of the resonator frequency imposed by the qubit metamaterial and the collective resonant coupling of eight qubits. The realized prototype represents a mesoscopic limit of naturally occurring spin ensembles and as such we demonstrate the AC-Zeeman shift of a resonant qubit ensemble. The studied system constitutes the implementation of a basic quantum metamaterial in the sense that many artificial atoms are coupled collectively to the quantized mode of a photon field. Manipulating the propagation of electromagnetic waves through sub-wavelength-sized artificial structures is the core function of metamaterials [1] , [2] , [3] . Resonant structures, such as split-ring resonators, play the role of artificial ‘atoms’ and shape the magnetic response. Superconducting metamaterials moved into the spotlight for their very low ohmic losses and the possibility of tuning their resonance frequency by exploiting the Josephson inductance [4] , [5] , [6] , [7] . Moreover, the nonlinear nature of the Josephson inductance enables the fabrication of truly artificial atoms [8] , [9] , [10] . Arrays of such superconducting quantum two-level systems (qubits) can be used for the implementation of a quantum metamaterial [11] , [12] . However, while natural atoms are identical, superconducting qubits are never the same exactly. For instance, the three-junction flux qubits [13] used in this work have a minimal energy-level spacing Δ, which is exponentially sensitive to the design parameters [14] . This makes the fabrication of qubits with similar specified properties very challenging. Moreover, in a linear qubit chain, which relies on the nearest-neighbour interaction, single off-resonant qubits act as defects and may destroy coherent modes. These drawbacks can be circumvented by using a common cavity for coupling the qubits one by one to a collective cavity mode [15] . The design of the quantum metamaterial presented here can be viewed as few-atom cavity quantum electrodynamics with artificial solid state atoms (see Fig. 1a ). 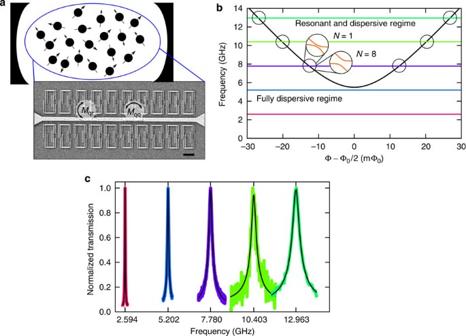Figure 1: A quantum metamaterial made of few artificial atoms in a cavity. (a) Coupling artificial atoms to the mode of an electromagnetic field is the main idea behind the concept of quantum metamaterials presented here. The scanning electron micrograph shows the central part of the coplanar wave guide resonator with 20 qubit rings situated between the central conductor line and the ground plane of the resonator; scale bar, 2 μm. The artificial atoms are much smaller than the wavelength of the transmitted signals, which is of the order of the length of the resonator (23 mm). Each qubit is individually coupled to the resonator by the mutual inductanceMqrand to its neighbour byMqq. Even thoughMqrandMqqare of the same order of magnitude, the effect of direct coupling between the qubits is inhibited by their strong dephasing (see Methods section). Therefore, the system effectively constitutesnmutually non-interacting spins coupled to the photon field of the resonator, similar to few-atom cavity quantum electrodynamics. (b) The level structure of the combined system of qubits and resonator. The horizontal lines (and their colour, as for the data traces in all subsequent figures) correspond to the modes of the resonator. The resonant phase shift expected at the crossings between qubits and resonator (encircled areas) is enhanced linearly by the number of qubitsN. The insets show the anticrossings forN=1 andN=8. In the fully dispersive regime, the metamaterial gives rise to a dispersive shift of the resonator frequency. (c) The transmission amplitude of the resonator at the fundamental mode frequency and the first four harmonics of the resonator. The black lines are fits to Lorentzians. The linewidthsκ/(2π) are 55.5, 216, 715, 950 and 1,400 kHz.κis the photon loss rate of the resonator. The widths of the curves are scaled over the frequency axis to a factor of 250 to ensure visibility over the full frequency range. The relative linewidth is to scale. Figure 1: A quantum metamaterial made of few artificial atoms in a cavity. ( a ) Coupling artificial atoms to the mode of an electromagnetic field is the main idea behind the concept of quantum metamaterials presented here. The scanning electron micrograph shows the central part of the coplanar wave guide resonator with 20 qubit rings situated between the central conductor line and the ground plane of the resonator; scale bar, 2 μm. The artificial atoms are much smaller than the wavelength of the transmitted signals, which is of the order of the length of the resonator (23 mm). Each qubit is individually coupled to the resonator by the mutual inductance M qr and to its neighbour by M qq . Even though M qr and M qq are of the same order of magnitude, the effect of direct coupling between the qubits is inhibited by their strong dephasing (see Methods section). Therefore, the system effectively constitutes n mutually non-interacting spins coupled to the photon field of the resonator, similar to few-atom cavity quantum electrodynamics. ( b ) The level structure of the combined system of qubits and resonator. The horizontal lines (and their colour, as for the data traces in all subsequent figures) correspond to the modes of the resonator. The resonant phase shift expected at the crossings between qubits and resonator (encircled areas) is enhanced linearly by the number of qubits N . The insets show the anticrossings for N =1 and N =8. In the fully dispersive regime, the metamaterial gives rise to a dispersive shift of the resonator frequency. ( c ) The transmission amplitude of the resonator at the fundamental mode frequency and the first four harmonics of the resonator. The black lines are fits to Lorentzians. The linewidths κ /(2 π ) are 55.5, 216, 715, 950 and 1,400 kHz. κ is the photon loss rate of the resonator. The widths of the curves are scaled over the frequency axis to a factor of 250 to ensure visibility over the full frequency range. The relative linewidth is to scale. Full size image Exploring the above ideas, we designed and fabricated a sample featuring 20 superconducting aluminium flux qubits embedded into a niobium microwave λ /2 cavity (see Fig. 1a ). For the used fabrication process, a spread of <20% in the energy gap Δ and of 5% in the persistent current I is achieved for the flux qubits [16] . The qubit–qubit nearest-neighbour coupling is designed to be negligibly small and the coupling of each qubit to the resonator is chosen as small enough, such that only the collective effects are expected to be visible. On resonance, when the level spacings of the qubits are equal to that of the resonator, the degeneracy between their states is lifted. This can be monitored by measuring the amplitude and phase of the microwaves transmitted at the resonator frequency. In the case of n mutually non-interacting qubits, an enhancement of the collective coupling by a factor of ( n ) 1/2 compared with the single-qubit case is expected [17] (see Fig. 1b ); this enhancement has been observed previously for three superconducting qubits [18] . However, the scalability of this effect for a larger number of qubits forming a macroscopic quantum system has not been tested. Here we use this effect in the resonant regime to identify three subensembles A, B and S of degenerate qubits and extract their average ensemble parameters. Interestingly, the system exhibits a time dependence, where the large ensemble S of eight qubits dissociates into the two smaller ones (A and B). In addition, we demonstrate the dispersive shift of the resonator frequency [19] , [20] by the qubits and show the tunabilty of the level structure of the quantum metamaterial by applying a coherent drive. One of the applications of our system is detecting and counting of single photons in the microwave frequency range [21] , [22] , [23] . Other proposals suggest the possibility to observe sudden phase switching [24] , quantum birefringence [25] and superradiant phase transitions [26] . Theoretical model In our system, the frequency spacing between the lowest two energy levels for the i th qubit is given by (ref. 13 ). By detuning the external magnetic flux Φ from the degeneracy point of half a flux quantum Φ 0 /2, an energy bias is provided. Thus, the energy splitting between the ground and the excited state of individual qubits can be controlled by changing the external magnetic field. Flux qubits are extremely anharmonic and therefore the influence of their higher energy levels can be ignored safely. The cavity is formed as a coplanar wave guide resonator with the fundamental mode at (see Supplementary Fig. 1 ). The coplanar wave guide resonator has higher harmonics with j =1,2,3,..., which are accessible through our measurement setup to j =5 (see Fig. 1c ). This feature permits the investigation of the resonant interaction at different frequencies. The photon field in the resonator is described by the creation and annihilation operators a † and a . The i th qubit Hamiltonian in the energy basis {| g i ›, | e i ›} can be expressed as , where are the Pauli matrices. The system of a single resonator mode coupled to n qubits is modelled by the Tavis–Cummings Hamiltonian [27] , where g ε , ij =(Δ i / E i ) g ij is the transverse coupling of one qubit to the resonator. The bare coupling g ij between qubit i and the resonator mode j can be calculated from the sample’s geometry. Numerical calculations for the used geometries reveal a mutual inductance M qr =(0.51±0.02) pH between a single qubit and the resonator and an inductance L r =(11±0.4) nH of the resonator (see Methods section). Subsequently, the coupling constant follows as . The dense packing of the flux qubits makes them less sensitive to local flux changes and prevents inhomogeneous coupling, which would be expected for larger types of superconducting qubits [28] . For large dephasing and resonant driving of the oscillator, we can use a semiclassical model for the description of the photon field, Γ φ is the dephasing rate of the qubits, f is the driving strength and is the detuning. We assume that the dephasing rate is the same for all qubits and because the driving is weak, we neglect terms of the order of |‹ a ›| 2 (see Methods section for further details). In the experiment, the phase φ of the transmission coefficient t of the resonator is monitored, t ∝ ‹ a ›=|‹ a ›| e iφ . If n qubits are in resonance, the stationary phase shift takes a simple form, The resonant regime The parameters of the qubit-resonator system are in the weak-coupling limit, where κ j ~ g ε,ij and Γ φ >> g ε,ij . Hence, single-qubit anticrossings are not resolvable from the base noise level. For n resonant qubits, an intermediate regime may be reached, when and . However, the vacuum Rabi splitting of a qubit-resonator anticrossing still cannot be resolved, because the decoherence of the qubits dominates over the coupling. Nevertheless, the signature of the anticrossing manifests itself in a dispersive shift of the resonance frequency [29] , [30] and a resulting phase shift. We performed the measurements in a dilution refrigerator with a nominal base temperature below 20 mK. The phase of the transmission through the sample at the harmonics of the resonator was recorded with a network analyser. A sufficiently small amplitude of the probe signal guaranteed that the average number of photons in the resonator was below unity. When the resonator is probed at its harmonics , two symmetric features appear most prominently in the third harmonic signal (see Fig. 2a ); they correspond to a resonant interaction between the qubits and the resonator. 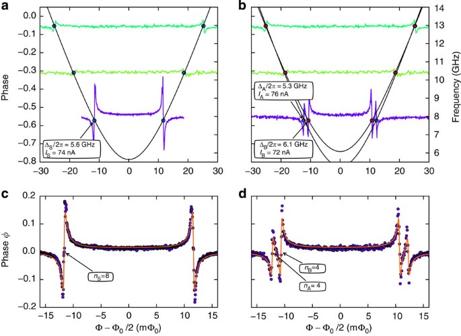Figure 2: The qubit metamaterial in the resonant regime. (a) The phase signal of the transmission through the system at the 3rd, 4th and 5th harmonic in dependence on the magnetic flux, which controls the transition frequencies of the qubits. The curves are separated in phase by an arbitrary offset. The rightyaxis presents the probe frequency of each curve (colour indicates the mode of the resonator) and also corresponds to the qubit frequencies of the effective parameter set S (black solid line). The extraction of the ensemble parameters results from the resonance points (closed circles). (b) Due to its sensitivity to charge fluctuations, the metamaterial possesses two stable states over time. Here, the parameters of the qubit system in the state of two resonant modes are extracted. (c) Quantitative analysis of the resonant mode between the qubits and the third harmonic mode of the resonator. The solid line shows a fit according to equation (2), which shows that ensemble S constitutes eight qubits. (d) The best fit for ensembles A and B yields four qubits each. Figure 2: The qubit metamaterial in the resonant regime. ( a ) The phase signal of the transmission through the system at the 3rd, 4th and 5th harmonic in dependence on the magnetic flux, which controls the transition frequencies of the qubits. The curves are separated in phase by an arbitrary offset. The right y axis presents the probe frequency of each curve (colour indicates the mode of the resonator) and also corresponds to the qubit frequencies of the effective parameter set S (black solid line). The extraction of the ensemble parameters results from the resonance points (closed circles). ( b ) Due to its sensitivity to charge fluctuations, the metamaterial possesses two stable states over time. Here, the parameters of the qubit system in the state of two resonant modes are extracted. ( c ) Quantitative analysis of the resonant mode between the qubits and the third harmonic mode of the resonator. The solid line shows a fit according to equation (2), which shows that ensemble S constitutes eight qubits. ( d ) The best fit for ensembles A and B yields four qubits each. Full size image To obtain the effective parameters of the qubits belonging to the ensemble that is responsible for the phase shift, the central frequencies of the resonances at harmonics are fitted as a function of the magnetic flux to the hyperbolic qubit spectrum E i (Δ i , ε i ) (see Fig. 2a ). The minimal energy-level spacing and persistent current are found to be Δ S /2 π =5.6 GHz and I S =(74±1) nA. Note that these are average values for the individual qubits taking part in the ensemble. Considering the fourth harmonic at frequency , the current of the standing wave at the centre of the resonator is expected to be zero and the voltage has maximum amplitude. Therefore, the interaction between the qubits and the resonator can only arise from capacitive rather than inductive coupling. We argue that the signature of crossing the qubit spectrum seen at the fourth harmonic is due to the relatively low ratio of Josephson energy to the charging energy of the Josephson junctions, leading to non-negligible capacitive coupling between the qubits and the resonator. Consequently, the qubits are sensitive to the charge fluctuations. This may cause low-frequency oscillations of the qubit energy leading to the observed splitting of the single resonance into two resonant modes over time, as shown in Fig. 2b (see Supplementary Note 1 and Supplementary Fig. 2 for further information). Each of the observed features ( Fig. 2a,b ) are stable over a timescale of ~10 3 s, which is much longer than the typical spectroscopy time of this experiment. The effective parameters of the ensembles responsible for the resulting two resonant modes A and B are Δ A /2 π =5.3 GHz, I A =(76±1) nA and Δ B /2 π =6.1 GHz, I B =(72±1) nA, respectively. The coupling of a single qubit to the third harmonic of the resonator follows as g i 3 /2 π =(1.2±0.1) MHz. The remaining unknown parameters of the system are the number of qubits n in the ensemble and the dephasing rate Γ ϕ . The dephasing is responsible for the width of the resonant mode, whereas the dispersive shift out of resonance is independent of the dephasing and depends solely on the number of qubits. Thus, n and Γ ϕ can be regarded as independent fitting parameters for the central region and for the periphery of the avoided level crossing, respectively. Notably, the magnitude of the resonator phase shift (equation (2)) depends linearly on n for a small number of qubits n . The best fit according to equation (2) for the most prominent resonant mode ( Fig. 2a ) between the qubit metamaterial and the third harmonic mode of the resonator yields n S =8 and Γ ϕ ,S =2 π × 53 MHz, as shown by the solid line in Fig. 2c . This dephasing rate corresponds to a phase coherence time of a few nanoseconds, as expected for flux qubits operated away from their degeneracy point. As the two separated resonant modes ( Fig. 2b ) are detuned from each other, they can be treated independently. The best fit of the measured data returns n A =4 and Γ ϕ ,A =2 π × 54 MHz, and n B =4 and Γ ϕ ,B =2 π × 41 MHz (see solid line in Fig. 2d ). The resonant mode of ensemble B is closer to its degeneracy point, which is consistent with a slightly lower dephasing rate. For each of the resonant modes, the number of participating qubits is half of that found for the single resonant mode. Therefore, we conclude that the ensemble of the single resonant mode (ensemble S, Fig. 2a,c ) is formed by the same qubits as ensembles A and B ( Fig. 2b,d ). The fully dispersive regime When all the minimal energy-level spacings Δ i are above the resonator frequency, no resonant interaction will occur. A frequency shift—the so-called dispersive dip—of the resonator is observed while tuning the magnetic field. It can be understood as a consequence of the AC-Zeeman shift, where each qubit shifts the cavity frequency by in a positive or negative direction, depending on its state [19] . If the system remains in the ground state at all times, the cavity shift depends solely on the qubit-resonator detuning. For frequencies below 5.3 GHz, the qubit metamaterial is in this fully dispersive regime, which can be analysed when probing the resonator at the fundamental mode frequency and at the second harmonic frequency . In this regime, the detuning between qubits and resonator δ ij is always higher than the dephasing Γ ϕ , which can be neglected. 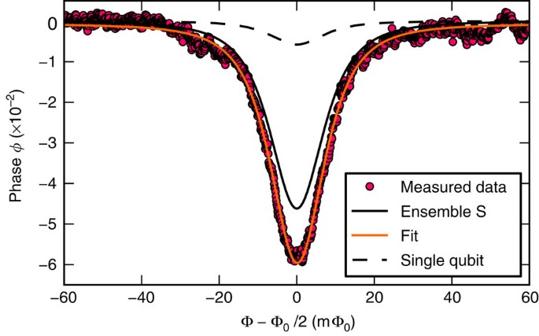Figure 3: Dispersive shift of the resonator frequency. For the fundamental mode of the resonator, the system is in the fully dispersive regime. The expected shifts for a single qubit (dashed line) and for the degenerate resonant subensemble S containing eight qubits (black solid line) are shown. A fit according to equation (2) with the number of qubits as free parameters and ensemble parameters S (orange solid line) yields an effective qubit numbern=10. Figure 3 shows the dispersive shift measured at the fundamental mode frequency . The expected shift induced by a single qubit is much weaker than the one actually observed. The theoretical dispersive shift for ensemble S does not account for the full magnitude of the shift. When fitted to equation (2) with the ensemble parameters S and n as a free parameter, the best fit is obtained for 10 qubits. The dominating influence on the dispersive shift arises from the qubits in the resonant modes, which possess a minimal detuning relative to the fundamental mode. The remaining qubits can have a higher minimal energy-level spacing resulting in a small contribution to the dispersive shift, which is proportional to 1/ E i 3 . Another explanation for their weak influence may be a very low persistent current or a very small gap, both resulting in a small coupling and therefore a small contribution to the dispersive shift. Nonetheless, the full extent of the dispersive shift is induced by all qubits in the metamaterial. Figure 3: Dispersive shift of the resonator frequency. For the fundamental mode of the resonator, the system is in the fully dispersive regime. The expected shifts for a single qubit (dashed line) and for the degenerate resonant subensemble S containing eight qubits (black solid line) are shown. A fit according to equation (2) with the number of qubits as free parameters and ensemble parameters S (orange solid line) yields an effective qubit number n =10. Full size image Tunability by a coherent drive Finally, to provide an evidence of the quantum nature of our system, we demonstrate the tunability of the dispersive shift by a photon number N j . By driving the metamaterial in an additional off-resonant mode j , its transition frequencies acquire a constant pull comparable to the AC-Zeeman shift occurring, for example, in natural spin ensembles. The shift is opposed on each qubit individually, the qubit frequencies are shifted in dependence on the sign of the qubit-resonator detuning δ ij to either higher or lower frequencies. The system under drive by N j photons follows (ref. 19 ). 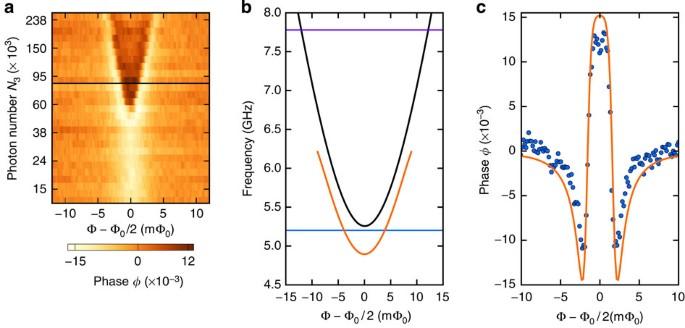Figure 4: The tunability of the qubit metamaterial by off-resonant driving by a coherent photon field. (a) The phase of the transmission (shading) in dependence on the photon numberN3at a frequency ofand a probe frequency of. At low driving strength, the metamaterial is in the fully dispersive regime, whereas at higher powers resonant modes appear. The metamaterial is in the state of two resonant modes. The horizontal line refers to the single trace depicted inc. (b) The level diagram of the system. The horizontal lines correspond to the harmonics of the resonator. In its initial condition, the qubit ensemble A is above the second harmonic frequency (black line). When driven at the third harmonic frequency, it is shifted below the second harmonic mode (orange line). (c) The resonant mode observed in the phase transmitted at the second harmonicfor a continuous drive at the third harmonic frequencywith a photon numberN3=85 × 103. The theoretical curve given by equation (2) of the resonant phase shift (solid line) between ensemble A and the second harmonic mode with no fitting parameters demonstrates the consistency of the extracted parameters. Figure 4a shows the transition from the dispersive regime to the resonant regime in the second harmonic mode. For a weak driving strength at a frequency of , ensemble A remains still above leaving the system in the fully dispersive regime (see Fig. 1b ) from which the coupling is extracted to be g i 2 =0.4 MHz (see Supplementary Note 2 and Supplementary Fig. 3 ). The resonant mode appearing at a photon number N 3 =85 × 10 3 is in good agreement with the theoretically expected one (see Fig. 4c ), showing that the parameters extracted are fully consistent with our expectations. Figure 4: The tunability of the qubit metamaterial by off-resonant driving by a coherent photon field. ( a ) The phase of the transmission (shading) in dependence on the photon number N 3 at a frequency of and a probe frequency of . At low driving strength, the metamaterial is in the fully dispersive regime, whereas at higher powers resonant modes appear. The metamaterial is in the state of two resonant modes. The horizontal line refers to the single trace depicted in c . ( b ) The level diagram of the system. The horizontal lines correspond to the harmonics of the resonator. In its initial condition, the qubit ensemble A is above the second harmonic frequency (black line). When driven at the third harmonic frequency, it is shifted below the second harmonic mode (orange line). ( c ) The resonant mode observed in the phase transmitted at the second harmonic for a continuous drive at the third harmonic frequency with a photon number N 3 =85 × 10 3 . The theoretical curve given by equation (2) of the resonant phase shift (solid line) between ensemble A and the second harmonic mode with no fitting parameters demonstrates the consistency of the extracted parameters. Full size image In conclusion, we have reported experiments and analysis of a prototype quantum metamaterial formed by 20 superconducting flux qubits. The studied system constitutes the implementation of a basic quantum metamaterial in the sense that many artificial atoms are coupled collectively to the quantized mode of a photon field. Despite the expected relatively large spread of the qubit parameters given by the exponential dependence on the energy gap Δ and the persistent current I of the qubits, the collective behaviour of the qubits is observed clearly. While all qubits give rise to a dispersive shift of the resonator frequency, the parameters of three different resonant ensembles of qubits are reconstructed by using their level crossing with the higher harmonics of the resonator. The quantitative analysis of the resonant modes reveals that two ensembles are formed by the collective interaction of four qubits each and the third ensemble is formed by eight qubits. The tunability of the ensembles by the AC-Zeeman shift has been demonstrated. Derivation of the qubit-resonator coupling The mutual inductance M qr =0.51±0.02 pH between a single qubit and the resonator and the inductance of the resonator L r =(11±0.4) nH are derived from the geometry of the sample. The uncertainty for the mutual inductance results from resolution of the micrograph from which the exact position and size of the qubit are extracted. The mutual inductance between qubits and resonator can also be easily estimated by the assumption of a rectangular loop with height h and length l placed at a distance x next to an infinite wire The qubit’s dimensions are l =1.6 μm and h =4.3 μm. Its distance to the central line of the resonator is 1.1 μm. This results in an inductance of M qr,e =0.51pH, which is identical to numerical calculations. In addition, our method has been experimentally validated using a single qubit embedded into an identical resonator with and κ 3 =0.46 MHz. The dimension and location of the qubit differs from the ones used in the metamaterial, the size of the qubit is l =4.6 μm and h =2.6 μm. It is placed at a distance x =1.8 μm, which results in a slightly higher mutual inductance M qr =(0.91±0.02) pH. The gap and the persistent current are Δ=3 GHz and I =(158±1) nA, determined in a two-tone spectroscopy experiment. The expected coupling is g qr /2 π =(4.7±0.3) MHz. Supplementary Figure 3 shows the transmission through the third harmonic of the resonator. As in the case for the metamaterial, two symmetric resonance points occur. The solid line shows a two-parameter fit with g qr and Γ ϕ as free parameters using equation (2) for n =1. The best fit is obtained for and Γ ϕ =2 π × 141 MHz. The experimental and theoretical values for the bare coupling are in very good agreement. The higher dephasing compared with the qubits in the metamaterial results from the larger detuning of the flux qubit from its degeneracy point. Quasiclassical equations of motion In this section, we will derive the equation of motion (1) for the radiation field of the oscillator mode. For the derivation, we will also allow qubit–qubit coupling, and show that as long as it is smaller than the dephasing rate Γ ϕ , it is of no relevance. The total Hamiltonian of the system is given by H T = H + H qq , where H is the Tavis–Cummings Hamiltonian, shown above, and H qq is the qubit–qubit coupling of the form We consider here nearest-neighbour coupling, with a coupling strength g qq . This gives us the following equations of motion with the qubit decay rate Γ 1 and the dephasing rate , where is the pure dephasing rate. We seek the solution of the equations of motion in the stationary limit, , and the semiclassical approximation ‹ σ k i a ›=‹ σ k i ›‹ a ›. In the zeroth order of g qq , we get Since the driving is very weak and |‹ a ›| 2 ≪ 1, we can neglect all terms of that order. This directly leads to the equation of motion (1), which we use to analyse the experiment. If we now try to understand the effect of the coupling terms, we see that in the semiclassical approximation we have and these terms can be neglected. Therefore, even with qubit–qubit coupling, we can assume ‹ σ z ›=−1. Using this assumption, we get the equation of motion From this, we get in first order of g qq Since Γ ϕ >> g qq , we see that the effect of qubit–qubit coupling can be neglected. How to cite this article: Macha, P. et al. Implementation of a quantum metamaterial using superconducting qubits. Nat. Commun. 5:5146 doi: 10.1038/ncomms6146 (2014).